Carrier density modulation in a germanium heterostructure by ferroelectric switching The development of non-volatile logic through direct coupling of spontaneous ferroelectric polarization with semiconductor charge carriers is nontrivial, with many issues, including epitaxial ferroelectric growth, demonstration of ferroelectric switching and measurable semiconductor modulation. Here we report a true ferroelectric field effect—carrier density modulation in an underlying Ge(001) substrate by switching of the ferroelectric polarization in epitaxial c -axis-oriented BaTiO 3 grown by molecular beam epitaxy. Using the density functional theory, we demonstrate that switching of BaTiO 3 polarization results in a large electric potential change in Ge. Aberration-corrected electron microscopy confirms BaTiO 3 tetragonality and the absence of any low-permittivity interlayer at the interface with Ge. The non-volatile, switchable nature of the single-domain out-of-plane ferroelectric polarization of BaTiO 3 is confirmed using piezoelectric force microscopy. The effect of the polarization switching on the conductivity of the underlying Ge is measured using microwave impedance microscopy, clearly demonstrating a ferroelectric field effect. Direct deposition of a ferroelectric oxide on a semiconductor typically results in a chemical reaction at the boundary between the two materials, yielding a thick amorphous interfacial layer and a polycrystalline ferroelectric film. The interfacial layer prevents the ferroelectric oxide from contacting the semiconductor in an atomically intimate manner and from having a measurable effect on the underlying semiconductor. Thus, the ferroelectric field-effect transistor (FeFET) has so far eluded development [1] . The conceptual simplicity of the FeFET architecture, combined with the large surface polarization charge density of a typical ferroelectric (~20 μC cm −2 ), an order of magnitude larger than what dielectrics can typically sustain, contribute to the obvious attraction of having a ferroelectric gate in a field-effect transistor. This seemingly straightforward approach has not yet worked because of the fundamental challenge of combining a ferroelectric oxide directly with a semiconductor without any interfacial reaction. To have a substantial effect on the semiconductor charge carrier density, the ferroelectric polarization charge must be as close to the transistor channel as possible. To achieve this proximity, one must ensure the highest-quality ferroelectric oxide/semiconductor interface, which requires heterogeneous epitaxy between the covalently bonded semiconductor and the ionically bonded oxide. In pioneering work, McKee et al. [2] were able to interface strontium titanate (STO) epitaxially with Si, thus opening up a path to integrate ferroelectric oxides such as lead zirconate titanate (PZT) and BaTiO 3 (BTO) with Si, using STO buffer layers [3] , [4] , [5] , [6] , [7] . However, it is nearly impossible to prevent formation of a low-permittivity SiO 2 layer at the STO–Si interface during subsequent deposition of the ferroelectric oxide, due to the very high reactivity of Si with oxygen. This intermediate layer prevents the ferroelectric polarization field from having any influence on the semiconductor, and also results in a depolarizing field that eventually kills the ferroelectric polarization [8] , [9] . An additional challenge for achieving functioning ferroelectric devices is that to modulate the semiconductor charge density by switching the polarization field, the latter must be aligned normal to the oxide/semiconductor interface. However, due to thermal expansion mismatch, for example, between BTO and Si, a residual in-plane tensile stress is present when the materials are cooled down after ferroelectric deposition. Hence, BTO tends to grow with its long tetragonal axis ( c axis), which is the direction of ferroelectric polarization, in the film plane. BTO has been epitaxially grown on Si using a variety of buffer layers but ferroelectric measurements show in-plane polarization [10] , [11] , [12] . Despite these difficulties, several groups have reported BTO grown on Si using various buffer layers, with the c axis normal to the interface [4] , [5] , [6] , [7] . Vaithyanathan et al. [5] demonstrated c -axis-oriented BTO growth on Si, but only after using a thick (30 nm), fully relaxed Ba 1− x Sr x TiO 3 (BST) layer to counteract the in-plane tensile stress due to the thermal expansion mismatch between BTO and Si. Niu et al. [6] reported c -axis-oriented BTO grown on Si using a 5-nm-thick STO buffer layer and showed a 0.75-V memory window in capacitance-voltage measurements for a 90-nm-thick film grown by pulsed laser deposition (PLD). Most recently, ferroelectric switching of perpendicular polarization without a bottom electrode has been demonstrated in epitaxial BTO films grown on STO-buffered Si for film thicknesses ranging from 8 to 40 nm with a smaller buffer thickness of 6 nm [7] . However, the presence of a low-permittivity 2-nm-thick interfacial SiO 2 layer required relatively high voltages to achieve switching. More importantly, the modulation of charge density in the semiconductor, in other words the ferroelectric field effect, was not demonstrated. Hence, one is faced with a dual challenge when trying to realize a FeFET on Si. On the one hand, most of the electric field is dropped across the low-permittivity SiO 2 layer, making it difficult to switch the ferroelectric. Conversely, even if switched, the polarization charge is removed from the channel because of the same SiO 2 layer. An alternative approach to integrating a ferroelectric directly on Si was proposed by Warusawithana et al. [13] , who grew ultrathin (<4 nm) strained STO directly on Si and showed using piezoelectric force microscopy (PFM) that the compressively strained STO film was ferroelectric. However, no measurements of the properties of Si were made, possibly due to the difficulty in dealing with device fabrication using such ultrathin films. There has recently been renewed interest in using Ge as a channel material [14] , [15] , [16] , [17] . As germanium is not as readily oxidized as silicon, one stands a much better chance of growing a ferroelectric oxide on Ge without any interfacial layer. Using Zintl templates several groups have made significant progress in interfacing BTO with Ge [18] , [19] , [20] , [21] . Merckling et al. [19] reported epitaxial BTO on thick Ge films grown on Si substrates: a ½-monolayer Ba template layer was used in analogy to the ½-monolayer Sr on Si used for STO on Si heteroepitaxy. Mixed c -axis-oriented and cubic phase growth was reported, and no measurements of the ferroelectricity or analysis of the interface structure were made. Because the BTO was grown using atomic oxygen, the interface was possibly oxidized with a buried GeO 2 layer that would be detrimental to direct coupling of the BTO polarization to Ge. We have recently demonstrated the fabrication of clean interfaces between Ge and BTO grown by molecular beam epitaxy (MBE), and between Ge and STO grown by atomic layer deposition [21] , [22] . We were able to infer the atomic structure of the BTO/Ge interface, but out-of-plane polarization was not demonstrated, due to thermal expansion mismatch. By inserting an ultrathin STO layer between BTO and Ge, one can impose compressive in-plane strain on BTO that can overcome tensile stress caused by the thermal expansion mismatch and thereby achieve BTO on Ge with out-of-plane polarization [5] ; a similar approach was recently used to grow BTO on GaAs. Ferroelectric switching of c -axis-oriented BTO on STO-buffered GaAs was demonstrated by Huang et al. [23] using preferentially oriented films with columnar crystallites, and by Contreras-Guerrero et al. [24] using flat epitaxial films. First-principles calculations To establish the feasibility of achieving the field effect in the presence of the STO layer, we performed first-principles calculations of the BTO/STO/Ge stack. Previous density functional theory (DFT) calculations have shown that BTO strained to STO remains ferroelectric even with only 1 unit cell of BTO present [25] , but the effect of polarization on the potential in the semiconductor layers beneath has not yet been considered. In simulations, we use a (001)-oriented eight-layer-thick p-type-doped Ge slab capped with three unit cells of STO on either side (for the STO–Ge interface we use the 2 × 1 model described in ref. 21 ). These are followed by seven-and-a-half unit cells of BTO with a TiO 2 -terminated surface facing vacuum. To satisfy the periodic boundary conditions, we use a large cell with mirror symmetry (see Supplementary Methods for details). The simulation cell and the macroscopic average of the electrostatic potential across it are shown in Fig. 1 . We find that there are two stable states of polarization. One, which we call P 1 , is essentially unpolarized and another, which we call P 2 , is polarized ‘down’ with Ti shifted away from the vacuum. In state P 1 , the few near-surface planes of BTO are polarized ‘down’ with the remainder of the layers being essentially flat. This is an artefact of the 2.8 nm thickness of BTO used in the calculation. The initial inward (‘down’) relaxation of Ti is induced by the surface and is well documented in TiO 2 (ref. 26 ). Of course, the local potential in the BTO bulk is totally symmetric. Therefore, polarization could be ‘up’ or ‘down’, but the ‘up’ polarization requires a head-to-head domain wall as one approaches the film surface. As the energy of such a wall, 0.11 J m −2 (ref. 27 ), is too high it is suppressed in ultrathin films. We will revisit this issue when discussing the electron microscopy results. We then examine the electrostatic potential for both polarization states. When comparing the difference in potential of the polarized and unpolarized heterostructures, we find a clear difference in electrostatic potential in the Ge layer as a result of switching between the two stable states of BTO polarization. This indicates that the presence of a high-permittivity STO layer does not interfere with a robust field effect. 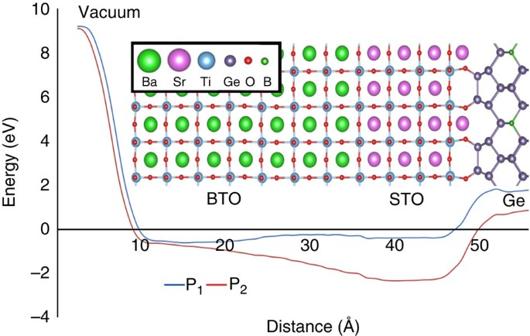Figure 1: Calculation supercell. The supercell used in the DFT calculations, consisting of vacuum, BTO, STO and B-doped Ge. The cell is mirrored on the other side (not shown). Note the recession of Ti from the surface, indicating polarization away from the BTO surface, and towards the BTO/STO interface. Below we show the macroscopic average of the plane-averaged electrostatic potential for the P1and P2states. Figure 1: Calculation supercell. The supercell used in the DFT calculations, consisting of vacuum, BTO, STO and B-doped Ge. The cell is mirrored on the other side (not shown). Note the recession of Ti from the surface, indicating polarization away from the BTO surface, and towards the BTO/STO interface. Below we show the macroscopic average of the plane-averaged electrostatic potential for the P 1 and P 2 states. Full size image Sample preparation and growth The Ge surface is prepared using a combination of wet-etching, oxygen plasma cleaning and annealing, resulting in a (2 × 1) reconstruction, low surface roughness and clear surface signal in the angle-resolved photoemission spectrum [28] . Prior to BTO growth, ½ monolayer of strontium is deposited to prevent germanium from oxidizing during the initial growth of the first five unit cells of STO at 200 °C. After increasing the temperature to 600 °C to crystallize the STO, BTO is co-deposited on the STO/Ge template at a temperature of 650 °C. A reflection-high-energy electron diffraction (RHEED) pattern of a 15-nm-thick film of BTO is shown in the inset of Fig. 2b . In situ X-ray photoelectron spectroscopy (XPS) measurements are carried out to determine the stoichiometry of the grown film ( Supplementary Fig. 1 ). 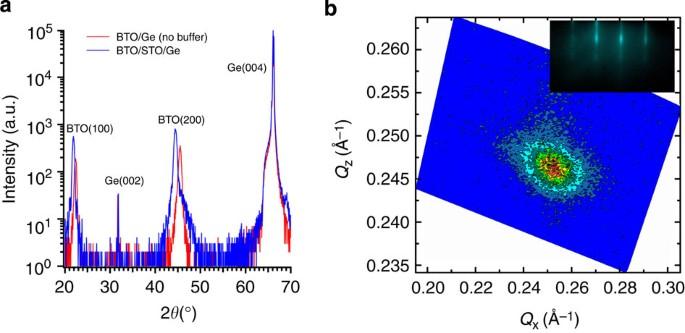Figure 2: Crystalline structure of BTO/STO/Ge. (a) X-ray diffraction 2θ−θscan of 16 nm BaTiO3epitaxially grown on Ge(001) substrate, with and without a 2 nm SrTiO3buffer layer. Without the buffer, the d-spacing corresponds to theaaxis of BTO directed out of plane. With the STO buffer, thecaxis of BTO is directed out of plane. (b) Reciprocal space map of the (103) Bragg reflection for BTO/STO/Ge. The centroid of the peak is consistent with a short in-plane axis and long out-of-plane axis. The inset shows a typical RHEED pattern for BTO/STO/Ge taken along the [110] azimuth showing good crystallinity and surface flatness. Figure 2: Crystalline structure of BTO/STO/Ge. ( a ) X-ray diffraction 2 θ − θ scan of 16 nm BaTiO 3 epitaxially grown on Ge(001) substrate, with and without a 2 nm SrTiO 3 buffer layer. Without the buffer, the d-spacing corresponds to the a axis of BTO directed out of plane. With the STO buffer, the c axis of BTO is directed out of plane. ( b ) Reciprocal space map of the (103) Bragg reflection for BTO/STO/Ge. The centroid of the peak is consistent with a short in-plane axis and long out-of-plane axis. The inset shows a typical RHEED pattern for BTO/STO/Ge taken along the [110] azimuth showing good crystallinity and surface flatness. Full size image Lattice constant determination using X-ray diffraction Films were characterized by X-ray diffraction performed on the BTO/Ge samples using a Philips X’Pert double-crystal diffractometer. Figure 2a shows symmetric θ −2 θ scans of a 160-Å-thick BTO film grown on Ge, both with and without a 20-Å-thick STO buffer layer. The BTO peaks correspond to a single orientation with an out-of-plane spacing of 4.06 Å for the film with the STO buffer, and 3.98 Å for the film without the buffer. This result clearly demonstrates the c -axis orientation for the STO-buffered sample compared with the a -axis orientation for the BTO layer grown directly on Ge. Figure 2b shows a reciprocal space map around the (103) Bragg reflection for the c -axis-oriented sample. The measured lattice constants after fitting with a two-dimensional Gaussian are a= 3.96 Å and c =4.06 Å. Rocking curve scans around the BTO 002 Bragg peak typically show a full-width at half-maximum of 0.5–0.8°. High-angle annular dark-field microscopy The crystalline quality of the BTO layer and the GeO 2 -free Ge surface are confirmed using cross-section aberration-corrected electron microscopy. Electron micrographs clearly reveal that the BTO layer is coherently strained to the partly relaxed STO buffer, with no dislocations visible along considerable lengths of the BTO/STO interface. Aberration-corrected images were recorded using a probe-corrected JEOL-ARM-200F, as shown in Fig. 3a . Individual Ti, Ge, Sr and Ba atomic-column locations can be identified in both bright-field and high-angle annular dark-field images, while Fourier transforms (diffractograms) of these images also confirm the tetragonality of the BTO with the longer c axis pointing out of the plane ( Fig. 3b ). Closer examination at higher magnification reveals that the Ti atomic columns close to the top of the BTO film are shifted downwards from the cell center, whereas in regions close to the STO film they are displaced slightly upwards ( Fig. 3c,d ). The ‘down’ polarization near the surface is in agreement with the theoretical prediction. 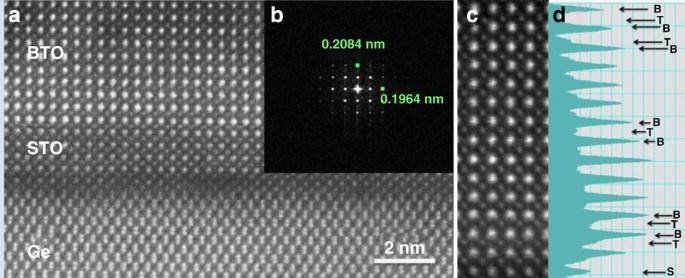Figure 3: Aberration-corrected electron microscopy. (a) High-angle annular dark-field (ADF) image of BTO/STO/Ge(001) heterostructure recorded with a 200-keV probe-corrected scanning transmission electron microscope. White spots correspond to positions of metal atoms. (b) Fourier transform of ADF image confirming tetragonality of the BTO layer. (c) Enlargement of the ADF image showing a region of the BTO film. (d) Corresponding line profile fromcshowing shifts in Ti atomic-column positions. Figure 3: Aberration-corrected electron microscopy. ( a ) High-angle annular dark-field (ADF) image of BTO/STO/Ge(001) heterostructure recorded with a 200-keV probe-corrected scanning transmission electron microscope. White spots correspond to positions of metal atoms. ( b ) Fourier transform of ADF image confirming tetragonality of the BTO layer. ( c ) Enlargement of the ADF image showing a region of the BTO film. ( d ) Corresponding line profile from c showing shifts in Ti atomic-column positions. Full size image Ferroelectricity confirmed by BE-PFM and BEPS The ferroelectric properties of the BTO layer were then tested using band-excitation PFM (BE-PFM) [29] , [30] . Results from a typical BE-PFM switching experiment are shown in Fig. 4a–c , where a 5 × 5-μm 2 square was initially poled with the tip held at −6 V, and a smaller 2.5 × 2.5-μm 2 square within the original square was then poled with the tip held at +4 V. The topography in Fig. 4a shows no change in the poled areas, suggesting no irreversible electrochemical reactions at the surface. At the same time, the vertical BE-PFM amplitude and phase images in Fig. 4b,c indicate clear and sharp boundaries, which are signatures of written ferroelectric domains, and largely obviate tip-injected surface charge effects dominating the contrast. This experiment also confirms that the BTO film outside the poled regions is monodomain, with polarization oriented towards the STO/Ge substrate in agreement with the theoretical predictions. 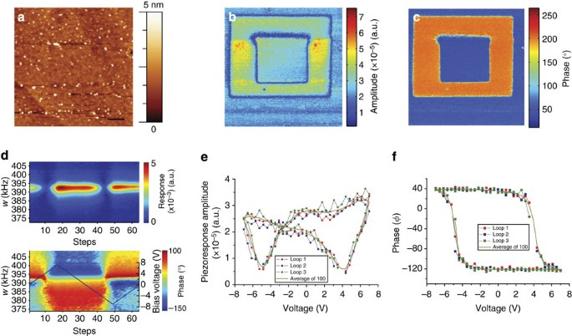Figure 4: PFM and voltage spectroscopy of BTO heterostructures. (a) Topography, (b) BE-PFM amplitude and (c) associated phase image after a box-in-box switching experiment on the BTO hetereostructure, showing clear ferroelectric switching (scale bar, 1 μm). A 5 × 5-μm2box was poled with the tip held at −6 V, and then a smaller box, 2.5 × 2.5 μm2, was subsequently scanned with the tip held at +4 V before the BE-PFM images were captured. Hundred hysteresis loops were then captured on the same film using BE spectroscopy. The average response is shown in the spectrograms indfor amplitude (above) and phase (below), with the applied d.c. waveform shown in blue. Selected amplitude and phase loops are shown ineandf, respectively, with the average loop shown as a solid line in olive. Figure 4: PFM and voltage spectroscopy of BTO heterostructures. ( a ) Topography, ( b ) BE-PFM amplitude and ( c ) associated phase image after a box-in-box switching experiment on the BTO hetereostructure, showing clear ferroelectric switching (scale bar, 1 μm). A 5 × 5-μm 2 box was poled with the tip held at −6 V, and then a smaller box, 2.5 × 2.5 μm 2 , was subsequently scanned with the tip held at +4 V before the BE-PFM images were captured. Hundred hysteresis loops were then captured on the same film using BE spectroscopy. The average response is shown in the spectrograms in d for amplitude (above) and phase (below), with the applied d.c. waveform shown in blue. Selected amplitude and phase loops are shown in e and f , respectively, with the average loop shown as a solid line in olive. Full size image To further characterize the ferroelectric properties of the BTO film, we carried out BE-piezoresponse spectroscopy measurements (BEPS [31] ), where the tip is placed at a particular position, a d.c. waveform is applied to the tip and simultaneously the BE response is captured to yield the system’s response. We performed a BEPS measurement on the BTO film across a 10 × 10 grid to yield a data set of 100 measurements in total; the average spectrogram of the response (amplitude and phase) is shown in Fig. 4d , with the d.c. waveform shown in the inset. Three selected responses at individual points from the 100 measurements, after fitting to a simple harmonic oscillator model, are shown in Fig. 4e,f (see also Supplementary Methods ; Supplementary Fig. 2 ). The average of 100 measurements is shown as a solid olive line. The amplitude curves clearly follow the expected butterfly-like hysteresis typical of ferroelectrics, while the phase loop appears to show a change somewhat <180°. The latter effect is probably due to a slight electrostatic contribution to the signal, which cannot be ruled out due to the lack of a bottom electrode in this sample. We also note that the coercive voltage appears largely symmetric with only a small offset, with values around +4 V and −5 V. Field effect demonstrated by microwave impedance microscopy Having demonstrated that the BTO layer is both polar and ferroelectric, we next turn to addressing the field effect. Due to the difficulty in fabricating BTO/Ge transistors, we utilize microwave impedance microscopy (MIM) to measure the conductivity of the underlying Ge [32] , [33] , [34] , [35] . MIM is a novel imaging tool used to spatially resolve the local permittivity and conductivity of materials [36] , [37] , [38] , and was employed to demonstrate the ferroelectric field effect in the BTO/STO–Ge heterostructures. Here the 1-GHz excitation signal is delivered to a specially designed cantilever probe [39] , and the evanescent wave from the tip apex, with a diameter of 20–100 nm, interacts with the sample underneath. The modulation of the carrier density at the ferroelectric–Ge interface results in an appreciable impedance change of the tip, which is readily detected by the MIM electronics. As shown schematically in Fig. 5a , a d.c. voltage of −4 V is also applied to the conductive MIM tip through a bias-tee to locally switch the BTO polarization. After a 20 × 20-μm 2 square was written, the d.c. bias was removed and a larger region concentric with the previous scan was then imaged by the same tip using PFM and MIM, both of which show clear contrast between the written and unwritten areas. The PFM contrast ( Fig. 5b ) again confirms that BTO polarization is reversed by a sufficiently large negative tip bias, with no corresponding topographic features. In Fig. 5c , the poled area shows substantially lower MIM real (MIM-Re) and slightly higher MIM imaginary (MIM-Im) signals than the intact region. Since neither the conductivity ( σ BTO =0) nor the first-order dielectric constant ( ε BTO ) of the BTO is affected by the polarization reversal, the MIM contrast must come solely from the underlying Ge layer accompanied by the poling process. We also confirmed that the PFM and MIM contrast is not observed for a smaller negative tip bias (| V tip |<4 V) or a positive bias up to +4 V, indicative of a ferroelectric switching process ( Supplementary Fig. 3 ). 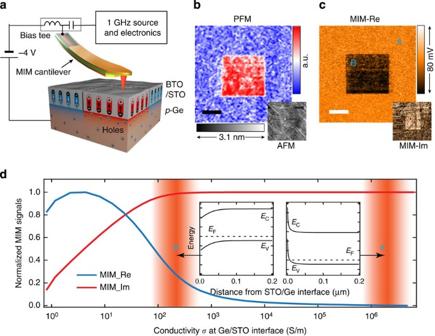Figure 5: Ferroelectric switching and electrical detection using microwave impedance microscopy. (a) Schematic diagram illustrating the measurement set-up and configuration of samples. A negative-biased conductive scanning probe makes downward to upward switching in ferroelectric polarization of the BTO layer, which modulates hole density at the BTO/p-Ge interface. PFM (b), AFM (bottom right corner inb), Microwave impedance microscopy (MIM) real part (c) and MIM imaginary part (bottom right corner inc) images acquired after writing a 20 × 20-μm2square by applying −4 V d.c. bias on the tip (scale bars, 10 μm). (d) Simulated MIM-Re (blue line) and MIM-Im (red line) signals as a function of conductivity at the BTO/Ge interface. Left and right insets, respectively, show band diagrams of Ge in regions A and B inc. Figure 5: Ferroelectric switching and electrical detection using microwave impedance microscopy. ( a ) Schematic diagram illustrating the measurement set-up and configuration of samples. A negative-biased conductive scanning probe makes downward to upward switching in ferroelectric polarization of the BTO layer, which modulates hole density at the BTO/p-Ge interface. PFM ( b ), AFM (bottom right corner in b ), Microwave impedance microscopy (MIM) real part ( c ) and MIM imaginary part (bottom right corner in c ) images acquired after writing a 20 × 20-μm 2 square by applying −4 V d.c. bias on the tip (scale bars, 10 μm). ( d ) Simulated MIM-Re (blue line) and MIM-Im (red line) signals as a function of conductivity at the BTO/Ge interface. Left and right insets, respectively, show band diagrams of Ge in regions A and B in c . Full size image Finite-element modelling [37] was performed to analyse the effect of carrier modulation in Ge on the MIM signals. Since the near-field interaction is highly dependent on the exact tip–sample contact condition, the simulation only serves as a qualitative guide to the experimental data. As shown in Fig. 5d , the MIM-Im signal, which is proportional to the tip-to-ground capacitance, rises monotonically with σ at the BTO/STO–Ge interface. On the other hand, the MIM-Re signal, which represents electrical loss within the probing volume, peaks at an intermediate σ Ge ( Supplementary Fig. 4 ). The higher MIM-Im and lower MIM-Re signals in the patterned square hence indicate a larger interfacial σ Ge than that of the unwritten area. As elaborated below, the MIM data clearly corroborate the conclusion of DFT calculations and scanning transmission electron microscope images that the polarization of the as-grown BTO layer is pointing towards the underlying Ge substrate. This as-grown ferroelectric polarization partially depletes holes in the p-type Ge (left inset of Fig. 5d ), giving rise to a lower interface conductivity than the bulk. After the BTO polarization is reversed by a sufficiently large negative tip bias, the energy bands drastically bend upwards (right inset of Fig. 5d ) and holes accumulate near the BTO/STO–Ge interface. As a result, σ Ge is much enhanced at the heterojunction, leading to the observed MIM contrast. To the best our knowledge, this is the first demonstration of carrier density modulation in semiconductors due to ferroelectric switching. In conclusion, the ferroelectric field effect is clearly demonstrated for highly crystalline c -axis-oriented BaTiO 3 , epitaxially grown on Ge(100) substrates using MBE via a thin (20 Å) SrTiO 3 buffer layer. The ferroelectric properties of the BTO layer and its effects on the underlying Ge are confirmed using PFM and MIM. Results of electron microscopy and PFM in regard to the microscopic nature of the effect can be well understood within the atomistic picture provided by the first-principles theory. Our results open the possibility of realizing a ferroelectric FET, leading to new non-volatile memories and low-power devices. Film deposition For film growth, p -type Ga-doped Ge(100) wafers from MTI Crystal Inc. ( ρ =0.05 Ω cm) that were diced into 10 × 10-mm 2 pieces are used as substrates. The samples are grown using a DCA M600 oxide MBE system with a base pressure of 3 × 10 −10 Torr and equipped with RHEED. Elemental Sr, Ba and Ti are evaporated using effusion cells. Growth rates are calibrated using a quartz crystal monitor to correspond to a deposition rate of one monolayer per minute, where a monolayer refers to the number of atoms per unit area in the unreconstructed, ideal Ge(100) surface. Growth rates are fine-tuned using a combination of XPS and the appearance of reconstruction spots in RHEED. Sample cleaning is performed by alternately dipping the sample in HCl and H 2 O 2 to remove surface contamination, prior to exposing the sample to oxygen plasma for 30 min at 300 W in situ [28] . After annealing the sample to remove the newly formed oxide layer from the Ge surface, ½ monolayer of strontium is deposited at a temperature of 500 °C. This critical Sr template prevents germanium from oxidizing during growth of the STO buffer. Five unit cells of STO are deposited onto this template by shuttering Sr and Ti effusion cells at a molecular oxygen pressure of 5.0 × 10 −7 Torr at 200 °C. To crystallize STO, the temperature is then increased to 550 °C (ramp rate: 30 °C min −1 ) and 600 °C (ramp rate: 20 °C min −1 ). After crystallization, the oxygen pressure is raised to 5.0 × 10 −6 Torr to co-deposit BTO on the STO/Ge template at a temperature of 650 °C. BTO crystallizes immediately as deposited. After growing the desired BTO thickness, the sample is then cooled to room temperature in oxygen (ramp rate: 10 °C min −1 ). Electron microscopy The probe-corrected electron microscopy was performed using a JEOL ARM-200F (camera length: 6 cm; probe convergence angle: 20 mrad; annular dark-field collection angle: 90~170 mrad) operated at 200 keV. Samples suitable for cross-section observation were prepared by standard mechanical polishing and dimpling, followed by argon-ion milling at ~2.5 keV to minimize surface amorphization. Density functional theory All calculations are done using DFT in the local density approximation using plane augmented-wave pseudopotentials as included in the Vienna Ab-Initio Simulation Package code [40] , [41] , [42] , [43] , [44] , [45] . We employ the Perdew–Zunger form of exchange-correlation potential [46] . We use the valence configuration 3p 6 4s 2 3d 2 for titanium, 5s 2 5p 6 6s 2 for barium and 2s 2 2p 4 for oxygen, and 3d 10 4s 2 4p 2 for germanium, 4s 2 4p 6 5s 2 for strontium and 2s 2 2p 1 for boron, and a 600 eV kinetic energy cutoff. For the Brillouin zone integration, we use a Monkhorst–Pack [47] 6 × 3 × 1 mesh for the BTO/STO/Ge heterostructure. For the BTO/STO heterostructure, the lateral unit cell is 3.98 Å, which is 1/√2 times the calculated lattice constant of Ge (5.63 Å). BE-PFM and spectroscopy BE-PFM and voltage spectroscopy are performed on a commercially available Asylum AFM platform (Cypher instrument) using PXI-based National Instruments data acquisition cards and in-house built software at CNMS, ORNL. Data analysis is performed on Matlab v2013b. The BE-PFM image is captured with a frequency bandwidth of 110 kHz centred at 385 kHz, with an applied a.c. voltage of 2.25 V to the tip at a scan rate of 1 Hz. The BEPS measurements are all carried out in the off-field state with a reading voltage of V a.c. =1.5 V. Microwave impedance microscopy The MIM in this work is based on a standard AFM platform (ParkAFM XE-70). The customized shielded cantilevers are commercially available from PrimeNano Inc. The excitation 1-GHz microwave signal is set at −20 dBm or 10 μW. The reflected signal carries the information of tip–sample admittance, which is detected by the electronics to form the MIM-Im and MIM-Re parts of the MIM images. Details of the MIM electronics can be found in ref. 37 . The finite-element analysis is performed using commercial software COMSOL4.3. How to cite this article: Ponath, P. et al. Carrier density modulation in a germanium heterostructure by ferroelectric switching. Nat. Commun. 6:6067 doi: 10.1038/ncomms7067 (2015).